Acetylacetone photodynamics at a seeded free-electron laser The first steps in photochemical processes, such as photosynthesis or animal vision, involve changes in electronic and geometric structure on extremely short time scales. Time-resolved photoelectron spectroscopy is a natural way to measure such changes, but has been hindered hitherto by limitations of available pulsed light sources in the vacuum-ultraviolet and soft X-ray spectral region, which have insufficient resolution in time and energy simultaneously. The unique combination of intensity, energy resolution, and femtosecond pulse duration of the FERMI-seeded free-electron laser can now provide exceptionally detailed information on photoexcitation–deexcitation and fragmentation in pump-probe experiments on the 50-femtosecond time scale. For the prototypical system acetylacetone we report here electron spectra measured as a function of time delay with enough spectral and time resolution to follow several photoexcited species through well-characterized individual steps, interpreted using state-of-the-art static and dynamics calculations. These results open the way for investigations of photochemical processes in unprecedented detail. It is a long sought-after goal to follow the dynamics of photoexcited molecular species on very short time scales using such tools as free-electron lasers (FELs) or high-harmonic generation (HHG). A colorful description of the ultimate objective is to call it the making of a “molecular movie”. Various attempts to characterize molecular dynamical processes on ultrashort time scales have been made at FELs, mostly with structural techniques such as photoelectron diffraction [1] , and X-ray diffraction/scattering [2] , [3] , [4] . Such methods require complex data manipulations and are insensitive to subtle differences in electronic structure, which albeit small can be vital to the process. A promising way to characterize the full electronic dynamics would be to look at valence photoelectron spectra in combination with ion yield spectra, to identify photochemical reaction pathways. Valence photoelectron spectra are directly informative of the electronic structure of the investigated species and can reveal variations in response to external parameters such as temperature change or photoexcitation. To observe the first stages of a chemical process using photoelectron spectra, picosecond (ps) or femtosecond (fs) time resolution is needed and the most suitable light sources to employ are FELs or HHG. Up to now this relatively simple approach has been hindered by the facts that at FELs the photon energy jitter is generally too large to give sufficiently resolved spectra without heavy data treatment and/or averaging over several time delays [5] , [6] , and with simple HHG the resolution is masked by the simultaneous presence of multiple harmonics. If harmonic filtering is employed, the resulting intensity is too low to follow subtle changes. A recent major breakthrough in this direction is represented by the newly built FERMI FEL at the Elettra facility, Trieste, Italy [7] . This seeded source provides pulses with negligible photon energy jitter, so photoemission spectra can be obtained with enough resolution to characterize very precisely ionization from different electronic states. The seeding scheme also provides an IR pulse which is very accurately synchronized to the FEL pulse, because it is derived from the Ti:Sa laser that drives the seed chain [8] , [9] , [10] . This IR pulse can be conditioned (change of delay, polarization, intensity; frequency doubling/tripling), and is conventionally named seed laser for users (SLU). Using the FERMI-seeded source in combination with the third harmonic of the SLU, 261 nm (4.75 eV), we have performed pump-probe experiments on a prototypical system, acetylacetone, which is a stable molecule used as solvent or as chelating agent [11] , [12] with potential environmental and medical applications [13] . The stable form in the gas phase at room temperature is the enol form stabilized by the intramolecular hydrogen bond; it can convert to the tautomeric keto form (see Fig. 1 for chemical formulas and possible fragmentation pathways) by proton transfer as a result of thermal activation or photoexcitation [14] , [15] , [16] , [17] . The photoexcitation/decay pattern of acetylacetone in the gas phase upon irradiation with a 266 nm wavelength has been reported in the literature [17] , [18] , [19] . Experimental evidence on the short time evolution remain however fragmentary, and conclusions rather tentative. A clearer picture was proposed by a theoretical study [17] . The molecule in the enolic form is initially promoted to the Franck–Condon (FC) region of the S 2 (ππ*) singlet state by 266 nm excitation. Decay to the S 1 (nπ*) state takes place in a short period by vibronic interaction, and finally the molecule relaxes to the T 1 (ππ*) triplet state by spin–orbit coupling (SOC). Rotational isomerization involving a breakage of the intramolecular O–H–O hydrogen bond and conversion of the C=C double bond to a single bond can then proceed from this state [16] , [17] leading to the keto form. A competitive process of OH elimination has also been shown to take place [18] from the lowest triplet T 1 (ππ*) state, with a time constant of 247 ± 43 ps after initial excitation to the singlet S 2 (ππ*) state. Another recent work [20] reports results on acetylacetone in different solvents, employing the same pump and transient spectroscopy as the main investigating tool. The excitation to the S 2 state and subsequent decay to the S 1 state are described, but the following step is assigned to the formation of a reaction product, namely a nonchelate enol, by rotamerization, which is concluded to be the dominant mechanism in solution. Fig. 1 Chemical formulas for the two tautomeric forms and possible fragmentation pathway Full size image Here, the main goal of our experiment is to follow the dynamics of the excited species in much greater detail than achieved previously, by exploiting the advanced characteristics of the FERMI-seeded source [7] , in particular the opportunity to obtain easy-to-read photoelectron spectra with good resolution and high statistics. We record valence electron and ion spectra with a magnetic bottle spectrometer [21] , [22] , [23] on the LDM (low density matter) beam line [24] , [25] , after pumping with the third harmonics of the SLU at 261 nm (estimated pulse duration 120–170 fs, energy per pulse up to 55 μJ) and probing with the fourth harmonic of FERMI at 19.23 eV (pulse duration ~100 fs, energy per pulse 40–60 μJ). The reported literature value for the excitation to the S 2 (ππ*) state is 266 nm, but the absorption peak is wide (ref. [17] and references therein), so that our pump induces the same transition. The negative values in the pump-probe delay scales in some of the figures represent FEL-only induced processes, recorded for reference purpose. The time evolution was followed up to 1.5 ps pump-probe delay with 50-fs steps and to 200 ps with larger steps. A clear picture of the evolution of the system is reached, showing that the photoexcitation to the S 2 (ππ*) (bright) state is followed by a conical intersection (CI) connecting with the S 1 (nπ*) (dark) state, and then the T 1 (ππ*) state is reached through ultrafast S 1 (nπ*)/T 2 (nπ*) crossing which is immediately followed by internal conversion to T 1 (ππ*). A minor pathway leading back to the ground state is also identified. Observed fragmentation yielding CH x species is related to the onset of the T 1 (ππ*) state formation. We believe this approach based on high-resolution valence spectra backed by high-level calculations is the ultimate way to shed light on fundamental, basic photo processes such as photosynthesis, photovoltaic energy production, and vision. General remarks A great asset of the experimental setup is that by simple changes of parameters it is possible to detect either electrons or ions with the same spectrometer and under exactly the same conditions in terms of pump-probe photon energies and delays. Let us note that the seed laser wavelength of the FEL, λ seed , is independent of that of the SLU, and can be tuned between 230 and 260 nm [7] in standard configuration. By changing transport mirrors, and making other modifications, it is also possible to cover the range 290 to 360 nm. The wavelength of the FEL, λ FEL , is then determined by setting its undulators at the desired harmonic n of λ seed ; for technical convenience we chose λ seed = 257.85 nm and set the undulators to n = 4, hence λ FEL = 64.46 nm. The residual time jitter between the FEL and the SLU is estimated at 6 fs [26] , [27] . Negative time delays in the horizontal scales for both ion and photoelectron spectra indicate delays where FEL ionization comes before the UV excitation pulse, i.e., FEL-only measurements. We have also run SLU-only spectra, to rule out the possibility of multiphoton processes induced by the pump. Two photons are sufficient to ionize the molecule, and ionization has been found to be negligible. Ion spectra The ion yield spectra for the most relevant ions are shown in Fig. 2 as functions of the pump-probe delay on time scales up to 5 and 200 ps. For each yield, the ratio of the integrated peak intensity between the initial value with FEL only and the values as a function of the pump-probe time delay are shown, to underline the relative variations. The dominant process revealed by the ion spectra is a fragmentation leading to production of the CH x + ion family ( x = 3, 2, 1, 0) within about 1 ps. All these ions could be produced by the photoionization of primary CH 3 . radicals at 19.23 eV, but C + can be formed this way only if the methyl radical is internally excited before ionization (the appearance energies from ground-state methyl radical are 9.8 eV for methyl ion, 15.1 eV for CH 2 + +H, 19.8 eV for CH + +2H, 15.3 eV for CH + +H 2 , 19.4 eV for C + +H 2 + H [28] ). Fig. 2 Ratios of integrated ion intensities. Top of panel: ratio of integrated ion intensities at a given delay to the integrated ion intensity at −1 ps (FEL only) for the fragments CH x + in the range 0–5 ps. Inset: same in the enlarged scale 0–200 ps. Bottom of panel: ratio of integrated ion intensities at a given delay to the integrated ion intensity at −1 ps (FEL only) for the fragments OH + and the parent ion as a function of pump-probe delay in the range 0–5 ps. Inset: same in the extended delay range 0–200 ps Full size image In Fig. 2 (top) we show the relative ion yields in the delay range 0–5 ps. The inset shows the trends in the extended delay range 0–200 ps. A large relative increase is evident in the production of the CH x + ion family. After 1–1.5 ps, the ion yields are substantially stable, up to 200 ps. In Fig. 2 (bottom) we show the OH + and the parent peak ion yields as a function of delay in the range 0–5 ps, and in the inset we show those in the extended delay range 0–200 ps. The OH + ion (appearance energy of OH . radical 13 eV [28] ) shows a very small increase in abundance during the first 2 ps after the pump, and then at longer delays shows a growing trend. Since the FEL photon energy is amply sufficient to ionize the OH radical, the observed trend is possibly compatible with the observation [18] that the neutral OH fragment is a major product after some hundreds of ps. Our results, to be discussed later in the paper, show that OH fragments are generated from the vibrationally hot ground state after internal conversion from S 1 or intersystem crossing from T 1 . The parent peak shows a continuous decrease over 1 ps, and then stabilizes. Photoelectron spectra Representative photoelectron spectra are shown in Fig. 3 , which is segmented into two parts. The binding energy range from 8.5 to 11 eV (electron kinetic energy range from 10.5 to 8 eV) shows photoionization of ground-state molecules, while the binding energy range from 3 to 8 eV shows photoionization of excited molecules. The two strongest bands, at 9.0 and 9.6 eV binding energy, are due to the enol form of the unexcited molecule [14] , [15] . The enol structure is the stable form at room temperature and the two main peaks correspond to molecular orbitals distributed on the π system and the oxygen lone pairs [14] . There are no significant changes in the valence photoelectron spectra of the ground state as a function of pump-probe delay. This observation rules out one of the possible photochemical processes, namely 261 nm photon-induced isomerization from the enol to the keto form (followed by relaxation back to the ground state): if that were to occur there would be two spectral features growing, corresponding to the + and − combinations of the oxygen lone pair orbitals in the keto form and including the band at 10.2 eV, while the first peak corresponding to the π system of the enol form should be depleted [14] , [15] . Fig. 3 Valence photoelectron spectra for a series of pump-probe delays Full size image While the photoelectron spectra corresponding to ionization of the ground state do not show any significant effect due to photoexcitation, the situation is very different for the low-binding energy region, where the spectral structures correspond to the ionization of excited species formed by the UV pump at 261 nm. We can identify three peaks in this region, at apparent binding energies of 4.64, 6.04, and 7.14 eV, each showing a different time evolution in the delay range 0–2 ps. To assign the three observed spectral features to the related excited states we have performed ab initio static and surface-hopping dynamics calculations. The relevant molecular structures optimized at the MS-CASPT2[10,10] level [29] , [30] are shown in Supplementary Fig. 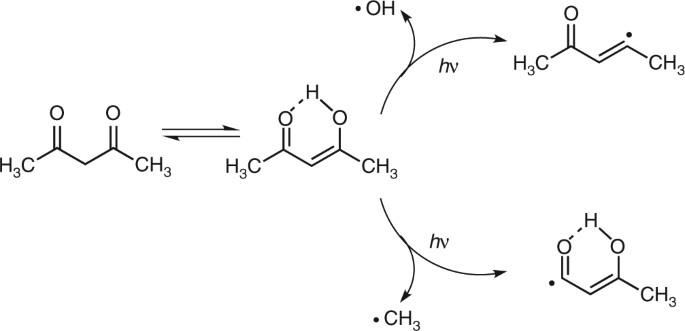Fig. 1 Chemical formulas for the two tautomeric forms and possible fragmentation pathway 1 (for Cartesian coordinates see Supplementary Table 1 ), while the corresponding excitation energies and mass-weighted distances from the reference ground state geometry (S 0min ) are given in Supplementary Tables 2 and 3 . Ionization energies (IE) also calculated at the MS-CASPT2[10,10] level are reported in Table 1 . 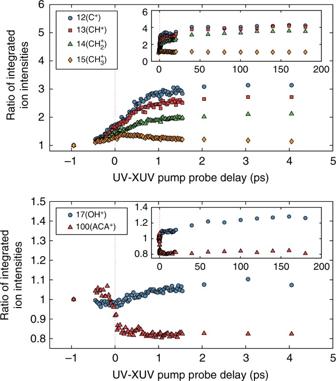Fig. 2 Ratios of integrated ion intensities. Top of panel: ratio of integrated ion intensities at a given delay to the integrated ion intensity at −1 ps (FEL only) for the fragments CHx+in the range 0–5 ps. Inset: same in the enlarged scale 0–200 ps. Bottom of panel: ratio of integrated ion intensities at a given delay to the integrated ion intensity at −1 ps (FEL only) for the fragments OH+and the parent ion as a function of pump-probe delay in the range 0–5 ps. Inset: same in the extended delay range 0–200 ps Table 1 Experimental and theoretical ionization energies (IE) of acetylacetone to the first ionic state (in eV) for the investigated transitions Full size table The calculated IE (D 0 −S 2 ) = 4.43 eV from the bright S 2 state at the S 0 minimum (S 0min ) geometry is in good agreement with the observed 4.64 eV energy of the lowest-lying peak (light blue curve). 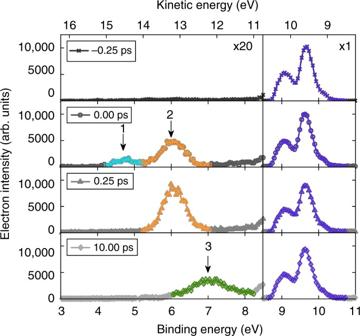Fig. 3 Valence photoelectron spectra for a series of pump-probe delays The equilibrium geometry of the S 1 state, S 1min , is geometrically close to the ground state minimum S 0min (Supplementary Table 3 ). At this geometry, the calculated ionization energy of 5.70 eV corresponds to the peak at 6.04 eV in the spectrum (orange curve). However, the peak at 6.04 eV has a more complex origin because at the S 1min geometry three electronic states, the singlet S 1 (nπ*) and triplets T 2 (nπ*) and T 1 (ππ*) are separated by only 0.1 eV. As the ground state of the cation is accidentally degenerate at this geometry with two states separated by only 0.02 eV, the IEs of all three states match the peak at 6.04 eV (Table 1 ). As for the third peak at 7.14 eV, the IE calculated for the minimum energy geometry of the T 1 (ππ*) state of 6.77 eV is in agreement with the experimental value (green curve). The minimum, T 1min , is highly deformed relative to the planar ground-state structure. At this geometry, the IE of the S 1 state (6.70 eV) also matches the experimental peak (Table 1 ). Therefore, the peaks at 6.04 and 7.14 eV may originate from different electronic states and can be attributed to ionizations from planar and distorted structures, respectively. Time evolution The transition from the S 2 (ππ*) singlet state to the S 1 (nπ*) state, with possible crossing to the T 2 (nπ*) and T 1 (ππ*) manifolds, and finally molecular deformation and relaxation to the T 1 (ππ*) state, are clearly reflected in the evolution over time of the three spectral features (Fig. 3 ) in this region corresponding to the ionization of the excited acetylacetone. 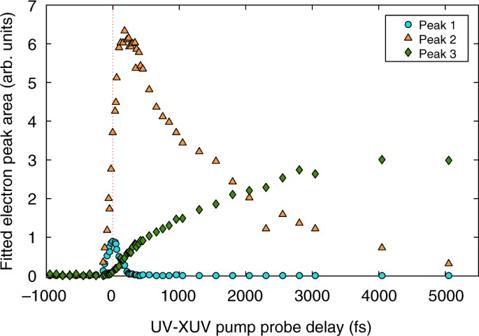Fig. 4 Experimental peak areas as a function of pump-probe delay. Given for peak 1 (4.64 eV), peak 2 (6.04 eV), and peak 3 (7.14 eV) Figure 4 shows fitted experimental peak areas intensities as a function of pump-probe delay time. 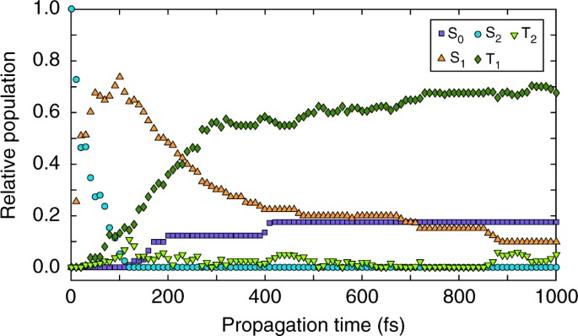Fig. 5 Average population of the adiabatic states. Given for the electronic ground state (S0), the two lowest singlet states, S2(ππ*) and S1(nπ*), and two triplet states, T2(nπ*) and T1(ππ*), obtained with CASSCF-based nonadiabatic dynamics simulations 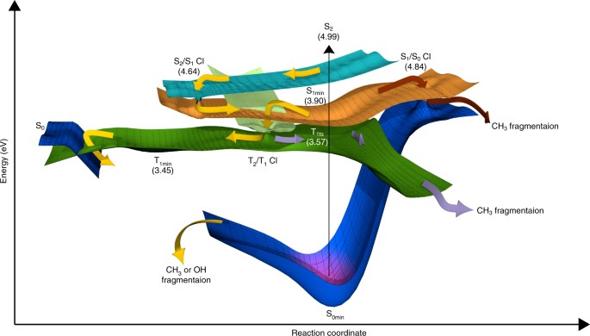Fig. 6 A schematic overview of the relaxation mechanism of acetylacetone. The ground state S0(darker blue), two singlet S2(ππ*) (light blue) and S1(nπ*) (orange), and two triplet T2(nπ*) (light green) and T1(ππ*) (green) states are shown. Excited state minima and minimum energy CIs (MECI) are indicated. Relative energies with respect to the electronic ground state minimum (S0min) are given. For details see Supplementary Tables1–3 The signal from the S 2 state (light blue curve) decreases rapidly and disappears at about 50 fs delay, the signal attributed to S 1 /T 2 /T 1 states arising from planar structures increases rapidly up to about 500 fs and then decreases, and the peak related to the T 1 state and non-planar structures increases up to about 3 ps and then becomes stable. Fig. 4 Experimental peak areas as a function of pump-probe delay. Given for peak 1 (4.64 eV), peak 2 (6.04 eV), and peak 3 (7.14 eV) Full size image To interpret the experimental trends, the calculated average population of all electronic states populated during the dynamics is shown in Fig. 5 . Note that the evolution of the electronic state populations shown in Fig. 5 and the dynamics of the three electron peaks, shown in Fig. 4 , are not directly comparable quantities, as three electronic states match the electronic peak centered at 6.04 eV (see Discussion section below). Fig. 5 Average population of the adiabatic states. Given for the electronic ground state (S 0 ), the two lowest singlet states, S 2 (ππ*) and S 1 (nπ*), and two triplet states, T 2 (nπ*) and T 1 (ππ*), obtained with CASSCF-based nonadiabatic dynamics simulations Full size image The 261 nm excitation promotes the molecule to the S 2 (ππ*) state. On the S 2 (ππ*) surface, the system initially evolves by elongation of the carbonyl C=O bond. The energy stabilization of the S 2 state along the C=O stretching coordinate leads to the CIs with the S 1 (nπ*) state. From Fig. 5 it is evident that the S 2 (ππ*)/S 1 (nπ*) CI seam is reached early in the dynamics as a complete population transfer to the S 1 (nπ*) state takes place within 100 fs, in agreement with the fast disappearance of the experimental peak at 4.64 eV. Once in the S 1 (nπ*) state, the trajectories split into three groups. Most trajectories (60%) reach the T 1 (ππ*) state through ultrafast S 1 (nπ*)/T 2 (nπ*) crossing which is immediately followed by internal conversion to T 1 (ππ*). T 2 (nπ*) is a doorway state and its population never reaches more than 10% (see Fig. 5 ). A smaller portion (15%) quickly passes from the S 1 (nπ*) state to the ground state, but this pathway is effectively closed after 400 fs. The remainder of trajectories stayed trapped in the S 1 (nπ*) state. To make a direct comparison with the time evolution of the experimental peaks we computed the IEs (Table 1 , Dynamics). Based on the results of dynamics simulations, IEs have been computed in time steps of 50 fs and averaged over all nonadiabatic trajectories residing in a given electronic state. From the IEs presented in Table 1 , one notices that, as long as the molecular ring is almost planar, the transfer of population S 1 → T 2 → T 1 will not be observed in the experimental spectrum as the third peak at 7.14 eV. This peak arises unequivocally from the T 1 state when the molecule deplanarizes. However, in the dynamics simulations, the rise of the peak at IE = 6.89 eV is exceedingly fast and occurs rapidly after crossing to the T 1 state. This suggests that either intersystem crossing is overestimated, causing excessively fast population transfer to the T 1 state, or that the molecule deforms too easily on the T 1 surface. By comparing CASSCF and CASPT2 SOC and energy differences between S 1 and the triplet states, we could rule out the first possibility, since we found no indication that the time scale of intersystem crossing is underestimated in the CASSCF-based dynamics. To investigate the second possibility, we computed the CASSCF and CASPT2 energy differences between T 1min and a planar transition state, i.e., T 1ts , that connects the two equivalent T 1min minima. Supplementary Fig. 2 shows that at the CASSCF level the energy difference is overestimated (0.37 eV) compared to the reference CASPT2 result (0.12 eV) causing indeed a fast deplanarization and early appearance of the peak at 7.14 eV in the dynamics. Additional information on the evolution of the system can be extracted from the ion spectra. To identify the electronic states from which fragmentation takes place, we computed the reaction paths for CH 3 and OH dissociation in the T 1 (ππ*) and S 1 (nπ*) states (Supplementary Figs. 3 and 4 ). In the relaxed scans computed at the MS-CASPT2[10,10] level, the barriers to dissociation should be compared to the S 2 (ππ*) excitation energy of 4.99 eV, which is the total amount of energy available to the system after photoexcitation. The potential energy profiles obtained on the T 1 state show that the dissociation of the methyl group starting from the planar T 1 (ππ*) minimum is possible. The barrier of E = 4.54 eV is significantly lower than either the one on the S 1 (nπ*) surface (~5.0 eV) or the one for the non-planar path on the T 1 (ππ*) surface (>5.0 eV). In contrast to the formation of methyl fragments, dissociation to form the OH radicals is not feasible from either of the excited states, implying that OH fragments are generated from the vibrationally hot ground state after internal conversion from S 1 or intersystem crossing from T 1 . Reaction path calculations on the ground electronic state show that dissociations to both OH and CH 3 , with barriers of 4.02 and 3.67 eV, respectively, are possible on this surface. The occurrence of CH 3 fragmentation only along the planar path on the T 1 (ππ*) surface suggests ultrafast population transfer to this state. In the experiment, there is a small difference in the rise of the ion (Fig. 2 ) and the 7.14 eV photoelectron curves (Fig. 3 , green line). The first reaches a plateau at ~1 ps whereas the second, arising from non-planar geometries in the T 1 (ππ*) state, becomes stable only after 2 ps. Thus, combined ion and photoelectron spectra, as well as static and dynamics calculations, hint at an S 1 /T 1 intersystem crossing in acetylacetone taking place on the picosecond or even subpicosecond time scale and leading to early appearance of CH 3 fragments. However, the possibility that CH 3 fragmentation occurs in the ground electronic state after ultrafast internal conversion from the S 1 state cannot be ruled out. The nature and time evolution of all states involved in the photodynamics are pictorially illustrated in Fig. 6 (see also Supplementary Fig. 6 ), which is to be considered a graphic summary of the behavior of the system. Schematically we illustrate the potential surfaces of the ground state and the two lowest singlet and triplet surfaces, as well as their crossing points, CIs and possible fragmentation pathways. Following the ultrafast internal conversion from the S 2 (ππ*) state (light blue) to the S 1 (nπ*) state (orange), three scenarios are possible: (i) Internal conversion from S 1 (nπ*) to S 0 involves passing through a high-lying seam of CIs (S 1 /S 0 CI at 4.84 eV) (Fig. 5 , brown arrows). The relative inaccessibility of this pathway is consistent with the slow disappearance of the S 1 (nπ*) peak at 6.04 eV. (ii) The dominant deactivation pathway leads to the population of the T 1 (ππ*) (green) state via the doorway state T 2 (nπ*) (light green). The high efficiency of intersystem crossing is due to the fact that for planar geometries close to S 1min the energy gap between the S 1 (nπ*), T 2 (nπ*) and T 1 (ππ*) states is very small. Norrish type-I methyl fragmentation is initiated upon crossing to the T 1 state along a planar reaction path (Fig. 6, violet arrows). The pathway is consistent with the observed fast increase in the ion yield of the CH x + fragments (Fig. 2 ). (iii) The system undergoes a roaming dynamics on the flat portion of the T 1 (ππ*) potential energy surface. On a longer time scale, geometry deformations on the T 1 state facilitate crossing to the electronic ground state from which both CH 3 and OH fragmentations are possible (Fig. 6, yellow arrows). Fig. 6 A schematic overview of the relaxation mechanism of acetylacetone. The ground state S 0 (darker blue), two singlet S 2 (ππ*) (light blue) and S 1 (nπ*) (orange), and two triplet T 2 (nπ*) (light green) and T 1 (ππ*) (green) states are shown. Excited state minima and minimum energy CIs (MECI) are indicated. Relative energies with respect to the electronic ground state minimum (S 0min ) are given. For details see Supplementary Tables 1 – 3 Full size image For comparison with previously reported results on the same system with a similar UV excitation as pump and different probe tools, we can make the following observations: In ref. [18] it was reported that the production of the OH fragment is related to the onset of formation of the T 1 state, with a time constant of 247 ps. However, from our data set we can clearly see that the formation of the T 1 state occurs much earlier, and it is achieved within few ps. This discrepancy is to be attributed to the fact that in ref. 18 electron diffraction was used to follow the evolution of the system, which cannot detect the small geometry changes between all excited states. Therefore, the onset of formation of OH should be attributed to the relaxation to the vibrationally hot ground state (see above Discussion). In ref. [19] the evolution from S 2 to S 1 was investigated with 266 nm pump–800 nm multiphoton probe in the delay range up to a few ps and low-kinetic energy electron spectra summed over several delays were shown. Ion yields were also recorded for some of the fragments, but not for the CH x family. A one-to-one spectral assignment for the various excited states as a function of pump-probe delay was not reported, and the transition to triplet states was not taken into consideration. Experimental The experiments were performed at the LDM beam line [24] , [25] of the FERMI FEL [7] , Trieste, Italy. The pump laser, denoted SLU (Seed Laser for Users), was set at the 3rd harmonic (261 nm) of the Ti:Sa base laser, horizontal polarization. The FEL beam was set at the fourth harmonic (19.23 eV) of the seed laser [8] , thus λ seed = 257.85 nm, λ FEL = 51.57 nm. Horizontal polarization was used. A highly-efficient, high-resolution magnetic bottle electron spectrometer with a retardation lens system of the Eland type [21] , [22] , [23] , similar to what was recently used at the AMO end station of the LCLS at Stanford, has been built and installed on LDM for the experiment. One of the latest development of our magnetic bottle technique allows detection of both electrons and ions at high collection efficiencies, retaining high energy resolution in particular for the electrons [22] , [23] , which was very important to match the superior performances of the FERMI light source [31] (see Supplementary Note 1 for a more detailed description of the spectrometer). Data treatment The raw electron/ion spectra were binned according to delay time and filtered so that shots with poor quality FEL light (low pulse energy) were rejected. The signal was summed and then normalized to the total FEL XUV energy in that bin as measured by the shot-to-shot energy detectors [32] . The electron time-of-flight spectra were then converted to kinetic energy using a variable width binning method, and a calibration derived from an ATI (above-threshold ionization) spectrum taken with the fundamental IR laser beam. The main peaks were referenced to the 2nd harmonic signal from ionization in He, which gives a constant spectral feature around 14 eV electron energy (see Supplementary Note 2 for more details). Computational static calculations Excitation energies were computed by performing a state-averaged multiconfigurational self-consistent field (SA-MCSCF) calculation including four singlet and two triplet states. The active space was selected by treating ten valence electrons as active electrons distributed among ten orbitals. The orbitals involved in the active space at the ground state minimum energy geometry are shown in Supplementary Fig. 5 . For ionization energies, a state-averaged calculation including two doublet states was performed using nine active electrons in ten orbitals. The energies were corrected by including the residual dynamical correlation contribution through multistate second order perturbation theory (MS-CASPT2) [29] . The cc-pVDZ basis set was used throughout the work. The Molcas [30] package was used for all calculations. Minimum energy CIs and singlet-triplet minimum crossing points were computed at the same MS-CASPT2[10,10] level using the sequential penalty constrained optimization method of Levine et al. [33] with default initial values of α = 0.025 Hartree and σ = 3.5. The harmonic-oscillator Wigner distribution for the nuclei was used to compute the ionization energies at the minima of the S 1 and T 1 states (Table 1 ) as well as the SOCs [34] . The computations were performed at the MS-CASPT2[10,10] level. When relaxing from the Franck–Condon region toward the minimum of the S 1 state, the system gains ~1.1 eV of kinetic energy, which is redistributed into molecular vibration. Accordingly, the Wigner distributions ware computed for an effective temperature of 600 K. Altogether 150 nuclear coordinates were sampled for each minimum. Deactivation pathways obtained from dynamics simulations and ion yield measurements were explored at the MS-CASPT2[10, 10] level. Linear interpolation in internal coordinates was used to connect optimized structures such as excited state minima and transition states. The intermediate geometries on these linearly interpolated paths were not optimized (rigid scans). Constrained MS-CASPT2[10, 10] optimizations along the C-CH 3 and C-OH stretching coordinates were performed to obtain relaxed scans of the potential energy for CH 3 and OH dissociation. Computational dynamics calculations Nonadiabatic molecular dynamics simulations have been performed using Tully’s fewest switches surface hopping algorithm [35] . Two sets of simulations have been performed. The first was based on the algebraic diagrammatic construction to second order (ADC(2)) method [36] , [37] , [38] , [39] and was restricted to singlet surfaces. The second, which was based on the CASSCF method and employed the same CAS-[10, 10] space as the one used in the static calculations, allowed switching between potential energy surfaces of different multiplicity. For the latter the SHARC program was used [40] , [41] , [42] . In SHARC calculations both nonadiabatic and SOC were included. SOC were calculated among four singlet (S 0 -S 3 ) and two triplet (T 1 , T 2 ) states. The surface hopping procedure was performed using the so-called diagonal states, i.e., states obtained by a diagonalization of the total Hamiltonian which includes SOC. The required gradients of the diagonal states were computed from the spin-free ones [41] . To facilitate the interpretation of the results, the populations of the electronic states shown in Fig. 5 have been transformed to the adiabatic basis. In total, 50 ADC(2) and 40 CASSCF trajectories have been launched from the S 2 (ππ*) state and propagated for 1 ps. Initial coordinates and velocities were generated from the vibrational ground state Wigner distribution which is the preferred sampling method for gas-phase systems of the size of acetylacetone [43] . Newton’s equations were integrated with time steps of τ1 = 0.5 fs whereas the time-dependent Schrödinger equation was integrated in time steps of τ2 = 5 ∙ 10–5 fs. The energy dependent decoherence scheme of Granucci and Persico with the default correction parameter of 0.1 Eh was employed in both types of simulations [44] . ADC(2) dynamics predicted an ultrafast S 2 → S 1 → S 0 deactivation along the C=O stretching and out-of-plane OH motion. CASSCF dynamics predicts a S 2 → S 1 → T 1 → S 0 decay that finds good agreement with the experiment. Data availability The data sets generated during and/or analyzed during the current study are available upon reasonable request from the corresponding author (M.N.P. ).